SynGAP isoforms exert opposing effects on synaptic strength Alternative promoter usage and alternative splicing enable diversification of the transcriptome. Here we demonstrate that the function of Synaptic GTPase-Activating Protein (SynGAP), a key synaptic protein, is determined by the combination of its amino-terminal sequence with its carboxy-terminal sequence. 5′ rapid amplification of cDNA ends and primer extension show that different N-terminal protein sequences arise through alternative promoter usage that are regulated by synaptic activity and postnatal age. Heterogeneity in C-terminal protein sequence arises through alternative splicing. Overexpression of SynGAP α1 versus α2 C-termini-containing proteins in hippocampal neurons has opposing effects on synaptic strength, decreasing and increasing miniature excitatory synaptic currents amplitude/frequency, respectively. The magnitude of this C-terminal-dependent effect is modulated by the N-terminal peptide sequence. This is the first demonstration that activity-dependent alternative promoter usage can change the function of a synaptic protein at excitatory synapses. Furthermore, the direction and degree of synaptic modulation exerted by different protein isoforms from a single gene locus is dependent on the combination of differential promoter usage and alternative splicing. The ability of neurons to dynamically regulate their response to changing inputs is essential for the accurate assembly and mature function of the nervous system. The induction and expression of neuronal plasticity is mediated by numerous mechanisms, many of which ultimately result in a change in the expression of synaptic proteins. For example, activity-dependent and developmental stage-dependent transcription factors [1] can use alternative promoters to create diversification of transcriptional regulation from a single locus [2] . Furthermore, functionally distinct proteins may be produced via regulated alternative splicing of messenger RNA [3] . Regulated protein trafficking then provides a mechanism to control the function of translated proteins. Many of the proteins that regulate neuronal plasticity are located in the postsynaptic density (PSD) [4] . SynGAP (Synaptic GTPase-Activating Protein) is a key PSD signalling enzyme that negatively regulates small G protein signalling downstream of glutamate receptor activation. SynGAP is physically linked to postsynaptic scaffold proteins (PSD-95, SAP-102) that bind to the N -methyl- D -aspartate receptor (NMDAR) forming a signalling complex with Ras family proteins and their effectors [5] , [6] . In mice, SynGAP has been shown to direct NMDAR-dependent alterations in synapse density, dendritic spine shape and synaptic physiology [6] , [7] , [8] . These outcomes are thought to be due largely to altered AMPA (α-amino-3-hydroxy-5-methyl-4-isoxazole propionic acid) receptor trafficking, which SynGAP both positively and negatively regulates [6] , [8] , [9] . Mice with reduced SynGAP expression show a decrease in hippocampal LTP and impaired spatial learning [6] , [10] . In humans, de novo mutations of SYNGAP have been identified in cases of non-syndromic mental retardation and autism spectrum disorder [11] , [12] . Syngap is a complex gene that gives rise to multiple protein isoforms with numerous functional domains [13] ( Fig. 1a ). Each isoform contains a central GAP domain that is responsible for enhancing the intrinsic GTPase activity of the small G proteins Ras and Rap. Three distinct isoforms of SynGAP, differing in their N-termini, have been reported although nothing is known about their origin or functional relevance [8] , [14] . SynGAPs A and B contain unique peptide sequences and a complete pleckstrin homology (PH) domain that may regulate lipid binding and protein–protein interactions [15] . SynGAP C is shorter, has no unique peptide sequence and lacks a complete pleckstrin homology domain. 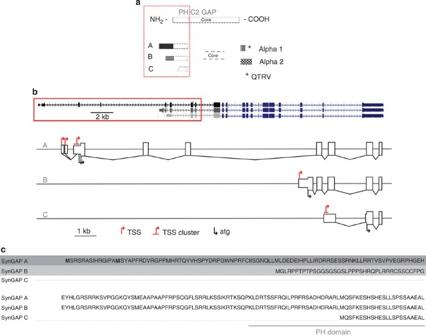Figure 1: Alternative SynGAP N-terminal peptides arise from distinct transcription starts sites. (a) A schematic diagram of potential SynGAP isoforms, which vary at both N-terminus (A, B and C) and C-terminus (α1 and α2 studied here, are shown; β and γ are not shown). (b) The exonic structure (blocks) of the threeSyngap5′ variantsA,BandCare illustrated on mouse genomic DNA (horizontal line, to scale in upper panel showing the full gene, scale is approximate in the expanded lower panel). Clusters of TSSs were found by RACE forSyngap AandCbut only one TSS was found forSyngap B. The transcription start sites ofSyngap Aare clustered approximately 10 kb upstream from those ofSyngap BandC. A thickening of the exon block indicates open reading frame that give rise to unique peptide sequences for SynGAP A and B, and a truncated N terminus for SynGAP C. Isoform-specific peptide sequences are shaded inc, the two alternative translation initiation codons (methionine, M) ofSyngap Aare highlighted by bold text, a horizontal line indicates the beginning of the pleckstrin homology (PH) domain. Figure 1: Alternative SynGAP N-terminal peptides arise from distinct transcription starts sites. ( a ) A schematic diagram of potential SynGAP isoforms, which vary at both N-terminus (A, B and C) and C-terminus (α1 and α2 studied here, are shown; β and γ are not shown). ( b ) The exonic structure (blocks) of the three Syngap 5′ variants A , B and C are illustrated on mouse genomic DNA (horizontal line, to scale in upper panel showing the full gene, scale is approximate in the expanded lower panel). Clusters of TSSs were found by RACE for Syngap A and C but only one TSS was found for Syngap B . The transcription start sites of Syngap A are clustered approximately 10 kb upstream from those of Syngap B and C . A thickening of the exon block indicates open reading frame that give rise to unique peptide sequences for SynGAP A and B, and a truncated N terminus for SynGAP C. Isoform-specific peptide sequences are shaded in c , the two alternative translation initiation codons (methionine, M) of Syngap A are highlighted by bold text, a horizontal line indicates the beginning of the pleckstrin homology (PH) domain. Full size image SynGAP also shows variation in protein sequence at the C-terminus, which arises from alternative splicing of Syngap mRNA and mediates SynGAP's interactions with other PSD proteins. The most studied C-terminal isoform is SynGAP α1, as it contains the PDZ-binding domain (QTRV) that mediates binding to scaffolding proteins of the PSD [6] , [7] . However, alternative splicing of Syngap mRNA leads to multiple isoforms (SynGAP α2, β, γ) that lack this PDZ-binding domain [13] . In particular, SynGAP α2 results from alternative splice junction selection and the insertion of a single frame-shifting base pair that removes the PDZ-binding domain and adds 48 unique amino acids at the C-terminus. The variability of SynGAP at both the N- and C-termini led us to hypothesize that the different isoforms have different functions. The role of particular domains have been previously examined, however, these studies have not examined how the N- and C-termini combine to alter SynGAP function. Therefore, we systematically investigated the functional consequences of expressing different full-length isoforms on spontaneous synaptic transmission, as well as the origin and regulation of the N-terminal variable regions. Our results demonstrate that the direction and degree of modulation exerted by SynGAP on spontaneous synaptic transmission is regulated by the precise combination of differential promoter usage and alternative splicing. SynGAP N-terminal variation results from use of alternative promoters Three different SynGAP N-terminal isoforms have been described that give rise to three distinct protein sequences, denoted SynGAP A–C [13] ( Fig. 1 ). We hypothesized that the expression of these N-terminal variants is under the control of different promoter regions and, hence, use unique sites for the initiation of transcription. We used 5′-rapid amplification of cDNA ends (5′ RACE) to clone full-length 5′ untranslated regions (UTRs) for each Syngap variant. Ten different clones were isolated by PCR using Syngap A-specific nested primers ( Supplementary Table S1 ), representing ten different putative transcription start sites (TSSs; Supplementary Table S1 ). Four different clones contained an open reading frame encoding a protein with the starting amino-acid sequence MSYAP-, corresponding to the protein previously reported [14] , which we now refer to as SynGAP A1. A further seven different clones displayed a longer open reading frame predicted to encode a protein with an additional 14 amino acids (alternative methionines emboldened in Fig. 1c ) at the N-terminus, which we now refer to as SynGAP A2. Nested primers specific for Syngap B yielded four clones of 371 bp ( Supplementary Table S1 ). These clones mapped to a single TSS (+10,515 bp, relative to ATG of Syngap A1 ). 5′ RACE with Syngap C -specific nested primers resulted in the isolation of eight different clones with 5′ UTRs ranging between 287 bp and 502 bp located between +11,164 bp and +11,379 bp (relative to ATG of Syngap A1 , Supplementary Table S1 ). Thus, only Syngap B uses a single TSS. These data are in agreement with recent genome-wide findings that transcription initiation can arise through the use of a cluster of TSSs (as we have found for Syngaps A and C) and is more common than the use of a classical single TSS ( Syngap B ) [16] . Therefore, SynGAP N-terminal isoforms arise through the use of distinct TSSs with those for Syngap s B and C located over 10 kb downstream of the Syngap A . To determine whether multiple promoters are present in the human gene, we performed a sequence comparison of the mouse genomic locus with that of human SYNGAP1 ( Supplementary Fig. S1 ). Bioinformatic analysis indicates that all residues of the SynGAP N-terminal isoforms are conserved between mouse, rat and human, despite containing no predicted functional moieties. We identified several regions of high similarity in introns, as well as exons, indicating functional significance for intronic sequences in regulating promoter activity. Examining data from the ENCODE project (ENCyclopedia Of DNA Elements), which aims to identify functional elements in the human genome sequence, it is apparent that the regions of high homology are also enriched in molecular hallmarks (such as histone modifications) of promoter and regulatory elements ( Supplementary Fig. S1 ). These enrichments occur in two clusters, one upstream of the Syngap A transcription start region and another upstream of the Syngap B and C start regions, suggesting that the different variants may be subject to independent transcriptional regulation. SynGAP N-terminus is regulated by synaptic activity and age To test whether Syngap is differentially regulated via different promoter regions, we examined the developmental and activity-dependent expression of Syngap variants in mouse cortical neurons using quantitative real-time reverse transcriptase (qRT)–PCR ( Fig. 2 ). Network activity was increased in dissociated neuronal cultures by applying the GABA A receptor antagonist bicuculline (Bic; 50 μM) to dis-inhibit synaptic activity. Syngap B and C were upregulated approximately twofold after 4 h of Bic treatment, whereas Syngap A was downregulated by 30% compared with vehicle-only control cultures ( Fig. 2b ). Total Syngap mRNA was unaltered indicating that Syngap A is the most abundant mRNA, as the decrease in Syngap A offsets the increase in Syngaps B and C . Application of the tetrodotoxin (TTX) blocked these changes in isoform expression, indicating that transcriptional regulation of Syngap is dependent on neuronal firing. No change was detected in Syngap levels after 1 h of treatment (data not shown). 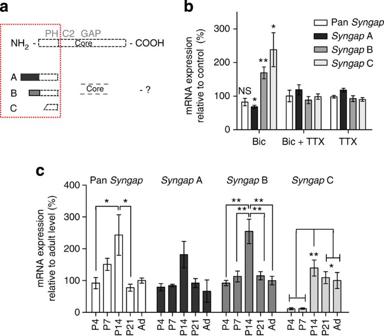Figure 2: Activity- and development-dependent regulation ofSyngapN-terminal variants. (a)Syngap5′ variant mRNA levels were examined by RT–PCR analysis. (b) Stimulation of synaptic activity in cultured forebrain neurons induces differential regulation ofSyngapmRNA variants (isoform-specific primers), despite causing no change in totalSyngaplevels (primers against the common core region). The approximate doubling ofSyngap BandCis offset by the approximately 30% decrease inSyngap A. Cultures were stimulated at DIV 10–12 with bicuculline and 4-aminopyridine (4-AP) for 4 h, bicuculline/4-AP stimulation is labelled as 'Bic'. Pairwise comparisons against control are indicated by asterisks over the bar. (c) RT–PCR analysis of mRNA levels in the developing postnatal mouse cortex reveals different temporal expression patterns ofSyngapvariants. Statistics are one-way ANOVA, followed bypost hocTukey tests. Statistically significant pairwise comparisons are indicated by linked bars,Syngap A, ANOVAP<0.05;post hoctestsP>0.05, *P<0.05, **P<0.01.n=3–5. Error bars represent s.e.m. Figure 2: Activity- and development-dependent regulation of Syngap N-terminal variants. ( a ) Syngap 5′ variant mRNA levels were examined by RT–PCR analysis. ( b ) Stimulation of synaptic activity in cultured forebrain neurons induces differential regulation of Syngap mRNA variants (isoform-specific primers), despite causing no change in total Syngap levels (primers against the common core region). The approximate doubling of Syngap B and C is offset by the approximately 30% decrease in Syngap A . Cultures were stimulated at DIV 10–12 with bicuculline and 4-aminopyridine (4-AP) for 4 h, bicuculline/4-AP stimulation is labelled as 'Bic'. Pairwise comparisons against control are indicated by asterisks over the bar. ( c ) RT–PCR analysis of mRNA levels in the developing postnatal mouse cortex reveals different temporal expression patterns of Syngap variants. Statistics are one-way ANOVA, followed by post hoc Tukey tests. Statistically significant pairwise comparisons are indicated by linked bars, Syngap A , ANOVA P <0.05; post hoc tests P >0.05, * P <0.05, ** P <0.01. n =3–5. Error bars represent s.e.m. Full size image Previous findings using antibodies that recognize all SynGAP isoforms indicated that SynGAP protein can be detected throughout postnatal cortical development with adult levels being reached by postnatal day (P)14 [17] . At the level of Syngap mRNA, primers that recognize all Syngap variants show that amounts peaked at the end of the second postnatal week and are significantly reduced by P21 ( Fig. 2c , analysis of variance (ANOVA), P =0.02, post hoc Tukey tests: P4 (92±17%) versus P14 (243±64%), P <0.05; P14 versus P21 (78±11%), P <0.05). However, each Syngap variant showed a distinct temporal profile of expression. Syngap A showed a pattern of regulation (ANOVA, P <0.05) but pairwise comparisons are not statistically significant by post hoc Tukey test, whereas Syngap B peaked at P14 (ANOVA, P =0.0013, P14 (254±38%) compared with P4 (92±8%), P7 (113±17%), P21 (115±13%), adult (100±14%), all post hoc tests P =<0.01). In contrast, Syngap C mRNA was expressed at low levels up to P7 (12±2%) but was subsequently upregulated approximately 12-fold by P14 (139±25%) and was not significantly downregulated in adulthood. Therefore, although Syngap B and C were similarly regulated by Bic treatment, they show different developmental profiles suggesting distinct (but possibly overlapping) mechanisms of regulation. SynGAP N- and C- terminal combinations The differential regulation of SynGAP N-termini suggested that transcriptional regulation could regulate SynGAP function. Previous work on SynGAP function had focused on one C-terminal isoform, SynGAP α1 (with a SynGAP C N-terminus), with very little known about the function of the α2 C-terminus. This leads to the obvious question of which combinations of N- and C-termini isoforms exist in neurons and if they can regulate synaptic function. Most Syngap sequences have been compiled from overlapping short clones, therefore, the in vivo linkage of N- and C-termini is not known. A full-length clone of SynGAP Cα1 has been isolated previously [18] and during a screen of a mouse cDNA library we isolated a full-length clone for SynGAP Aα2 ( Supplementary Information ). To determine if SynGAP α1 and α2 are present in neurons, we used isoform-specific antibodies to show that both C-terminal isoforms are expressed in the adult hippocampus and cortex ( Fig. 3 ). Western blot analysis revealed a doublet for both SynGAP α1 and SynGAP α2 around 130 kDa but with the upper bands of α2 isoforms separating at a higher molecular weight ( Fig. 3a ), reflecting the longer peptide sequence at the C-terminus of SynGAP α2 relative to SynGAP α1. The presence of multiple bands further suggests that there is heterogeneity in the N- and C-terminal sequences that combine to generate a SynGAP protein. Mass spectrometric analysis of purified PSDs confirmed that both SynGAP α1 and α2 are present at excitatory synapse indicating that α2 containing isoforms localize to PSDs despite lacking the QTRV sequence that binds to PDZ domains ( Supplementary Table S2 ). 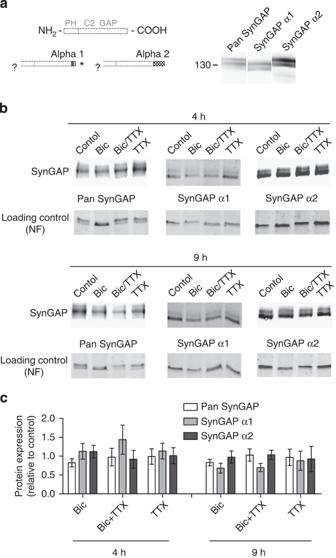Figure 3: Expression of C-terminal isoforms SynGAP α1 and α2 are not regulated by synaptic activity. (a) Mouse hippocampal homogenate was probed with antibodies against a region common to all isoforms (pan SynGAP), SynGAP α1 and SynGAP α2. To allow direct comparison of electrophoretic migration between isoforms, a single-protein-bearing nitrocellulose lane was cut into strips and each strip incubated separately with antibodies, then re-assembled. Antibodies to SynGAPα1 or SynGAPα2 each label doublets but of distinct molecular weight, consistent with the predicted difference in the length of their C-terminus. Furthermore, the distinct doublets suggest each C-terminus can be combined with several N-termini. (b,c) Stimulation of synaptic activity in cultured forebrain neurons does not affect the expression level of different SynGAP C-terminal isoforms. Cultures were stimulated at DIV 10–12 with bicuculline and 4-AP for 4 and 9 h, bicuculline/4-AP stimulation is labelled as 'Bic'. Four experimental replicates were performed. Error bars represent s.e.m. Figure 3: Expression of C-terminal isoforms SynGAP α1 and α2 are not regulated by synaptic activity. ( a ) Mouse hippocampal homogenate was probed with antibodies against a region common to all isoforms (pan SynGAP), SynGAP α1 and SynGAP α2. To allow direct comparison of electrophoretic migration between isoforms, a single-protein-bearing nitrocellulose lane was cut into strips and each strip incubated separately with antibodies, then re-assembled. Antibodies to SynGAPα1 or SynGAPα2 each label doublets but of distinct molecular weight, consistent with the predicted difference in the length of their C-terminus. Furthermore, the distinct doublets suggest each C-terminus can be combined with several N-termini. ( b , c ) Stimulation of synaptic activity in cultured forebrain neurons does not affect the expression level of different SynGAP C-terminal isoforms. Cultures were stimulated at DIV 10–12 with bicuculline and 4-AP for 4 and 9 h, bicuculline/4-AP stimulation is labelled as 'Bic'. Four experimental replicates were performed. Error bars represent s.e.m. Full size image If there was absolute linkage between particular N- and C-termini one would expect that regulation of the C-termini would mirror that of specific N-termini. However, unlike what was observed for the N-terminal isoforms, stimulation of neuronal cultures with Bic for either 4 or 9 h did not lead to any change in SynGAP α1 and α2 protein levels (SynGAP protein levels were assayed instead of mRNA as SynGAP α1 and α2 mRNAs differ by only 1 bp), further supporting that multiple combinations of N- and C-termini exist ( Fig. 3b,c ). These data indicate that multiple SynGAP proteins are generated from a single gene, suggesting that SynGAP may have several functional roles at synapses. Opposing effects of SynGAP isoforms on synaptic function To test the hypothesis that promoter selection combined with alternative splicing to generate SynGAP isoforms with distinct effects on synaptic function, we transfected forebrain neurons with plasmids containing full-length cDNA clones of Syngap with all combinations of N-termini (A, B and C) and C-termini (α1 and α2) along with enhanced green fluorescent protein (eGFP). In these and all subsequent experiments where SynGAP A was used it was always SynGAP A1 not A2 (see Fig. 1 and Supplementary Table S1 ). Whole-cell patch-clamp recordings from fluorescent neurons ( Fig. 4 ) revealed heterogeneity in the proportion of cells that exhibited AMPA receptor-mediated miniature excitatory synaptic currents (mEPSCs). We categorized neurons depending on whether mEPSCs were present or not; neurons lacking any mEPSCs were termed 'silent' cells ( Fig. 4b ). Importantly, silent cells were viable and healthy as they were able to fire action potentials (in the absence of TTX) and did not differ from controls in their holding currents or gross morphology (data not shown). To assess whether the apparent silencing effect was due to the particular SynGAP construct transfected, we examined the proportion of silent cells in each group ( Fig. 4c ). We found marked differences in the percentage of silent cells across all constructs (F (6, 37.4) =3.96, P =0.004). The majority (72.5%) of neurons transfected with SynGAP Aα1 lacked any mEPSCs, compared with a minority (10.5%) of control neurons. Only 45% of neurons expressing SynGAP Bα1 and 44.7% expressing Cα1 were silent. In contrast to the expression of SynGAP α1 isoforms, the expression of SynGAP α2 isoforms did not increase the percentage of silent cells. The proportion of silent SynGAP Aα2- and SynGAP Cα2-expressing cells (14.3 and 5%) was comparable to control (10.5%). For SynGAP Bα2, none of the transfected neurons lacked mEPSCs. Comparison of the distribution of mEPSCs to the control quartiles ( Fig. 4d ) showed that SynGAP Aα2 follows the control distribution very closely with approximately 25% of values in each category. In contrast, the distributions of SynGAP Bα2 and Cα2 mEPSCs had a reduced proportion of events in the small (20% and 16%, respectively) and medium (19% and 20%, respectively) ranges and an increase in events in the largest category (36% and 37%, respectively). Furthermore, the levels of silence observed in cells transfected with Syngap A α1 and A α2 are comparable between wild-type cells and in Syngap − / − cells, indicating that the endogenous expression of a range of SynGAP isoforms does not impact on the data we have obtained that show isoform-specific effects on mEPSC amplitudes and frequencies ( Fig. 4e ). 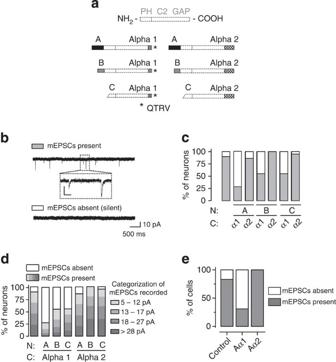Figure 4: Expression of different SynGAP isoforms alters the proportion of neurons exhibiting mEPSCs. (a) The effect of different SynGAP isoforms on synaptic transmission was assessed by recording mEPSCs from neurons expressing one of six individual isoforms composed of an N-terminus of A, B or C linked to either an α1 or α2 C-terminus. (b,c) Neurons were categorized as either having mEPSCs (top trace inband grey bar inc; inset scale: 10 pA and 25 ms) or not (silent, lower trace inband white bar inc). Data are displayed as a percentage of cells recorded for each construct. The percentage of neurons categorized as silent is as follows: control=10.5%,n=76; SynGAP Aα1=72.6%,n=62; SynGAP Bα1=45%,n=63; SynGAP Cα1=44.7%,n=40; SynGAP Aα2=14.3%,n=31; SynGAP Bα2=0%,n=38; and SynGAP Cα-2=5%,n=20. Data are from 18 transfections from 15 cultures, analysed using a generalized linear mixed model (F(6, 37.4)=3.96,P=0.004). (d) Data from all transfected cells are plotted to illustrate the proportion of silent cells (white bars), and mEPSCs of particular amplitude ranges (shaded bars). To illustrate the distribution of events, those from non-silent cells were further subdivided into four amplitude ranges, which were defined by the quartiles of the control event distribution. Number of events (n) from number of cells (N); eGFP,n=7,731,N=27; SynGAP Aα1,n=2756,N=11; SynGAP Bα1,n=2,664,N=10; SynGAP Cα1,n=4,044,N=17; SynGAP Aα2,n=6,712,N=23; SynGAP Bα2n=6,824,N=21; SynGAP Cα2,n=4383,N=15. Data are from 18 transfections from 15 separate cultures. (e) SynGAP−/−forebrain neurons were transfected with SynGAP Aα1 or Aα2. Neurons were categorized as being silent (white bars) or having mEPSCs (shaded bars). Data are displayed as a percentage of cells recorded for each construct. The percentage of neurons categorized as silent is as follows: GFP only=17%,n=29; SynGAP Aα1=69%,n=29,P<0.0001; SynGAP Aα2=0%,n=12. Populationχ2test,P<0.0001. Error bars represent s.e.m. Figure 4: Expression of different SynGAP isoforms alters the proportion of neurons exhibiting mEPSCs. ( a ) The effect of different SynGAP isoforms on synaptic transmission was assessed by recording mEPSCs from neurons expressing one of six individual isoforms composed of an N-terminus of A, B or C linked to either an α1 or α2 C-terminus. ( b , c ) Neurons were categorized as either having mEPSCs (top trace in b and grey bar in c ; inset scale: 10 pA and 25 ms) or not (silent, lower trace in b and white bar in c ). Data are displayed as a percentage of cells recorded for each construct. The percentage of neurons categorized as silent is as follows: control=10.5%, n =76; SynGAP Aα1=72.6%, n =62; SynGAP Bα1=45%, n =63; SynGAP Cα1=44.7%, n =40; SynGAP Aα2=14.3%, n =31; SynGAP Bα2=0%, n =38; and SynGAP Cα-2=5%, n =20. Data are from 18 transfections from 15 cultures, analysed using a generalized linear mixed model (F (6, 37.4 )=3.96, P =0.004). ( d ) Data from all transfected cells are plotted to illustrate the proportion of silent cells (white bars), and mEPSCs of particular amplitude ranges (shaded bars). To illustrate the distribution of events, those from non-silent cells were further subdivided into four amplitude ranges, which were defined by the quartiles of the control event distribution. Number of events ( n ) from number of cells ( N ); eGFP, n =7,731, N =27; SynGAP Aα1, n =2756, N =11; SynGAP Bα1, n =2,664, N =10; SynGAP Cα1, n =4,044, N =17; SynGAP Aα2, n =6,712, N =23; SynGAP Bα2 n =6,824, N =21; SynGAP Cα2, n =4383, N =15. Data are from 18 transfections from 15 separate cultures. ( e ) SynGAP −/− forebrain neurons were transfected with SynGAP Aα1 or Aα2. Neurons were categorized as being silent (white bars) or having mEPSCs (shaded bars). Data are displayed as a percentage of cells recorded for each construct. The percentage of neurons categorized as silent is as follows: GFP only=17%, n =29; SynGAP Aα1=69%, n =29, P <0.0001; SynGAP Aα2=0%, n =12. Population χ 2 test, P <0.0001. Error bars represent s.e.m. Full size image To ensure that the differential effects of SynGAP isoform expression on synaptic function did not simply arise from a mislocalization of particular isoforms, we transfected Syngap − / − hippocampal neurons with each SynGAP isoform and performed immunofluorescence with an antibody that recognizes all SynGAP isoforms. 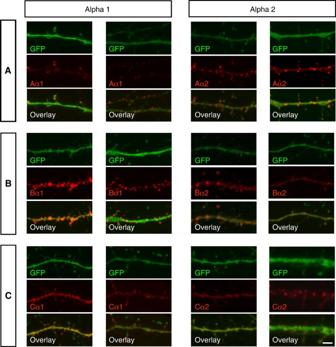Figure 5: SynGAP isoforms localize to dendrites and dendritic spines. Different SynGAP isoforms display different dendritic localization patterns but all are capable of reaching the postsynaptic compartment. SynGAP−/−forebrain neurons transfected with individual SynGAP isoforms were probed with an antibody against all SynGAP isoforms. Examples of dendritic sections from two different neurons are shown for each isoform. GFP (green) and SynGAP labelling (red) are shown above the overlaid images. Scale bar, 2 μm. Dendritic protein expression levels of various SynGAP isoforms expressed in SynGAP−/−neurons were quantified by semi-quantitative confocal microscopy (Supplementary Fig. S2). Figure 5 shows that all isoforms localize to dendrites and spines. Furthermore, there was no correlation between effect strength and isoform expression level ( Supplementary Fig. S2 ), indicating that the overexpression of SynGAP isoforms per se does not alter synaptic function in a non-specific manner. This is particularly highlighted by SynGAP Aα2, which had no effect on the proportion of silent cells or the profiles of the mEPSCs recorded, indicating that the effects of other isoforms are not due to non-specific effects of transfection or overexpression. Figure 5: SynGAP isoforms localize to dendrites and dendritic spines. Different SynGAP isoforms display different dendritic localization patterns but all are capable of reaching the postsynaptic compartment. SynGAP −/− forebrain neurons transfected with individual SynGAP isoforms were probed with an antibody against all SynGAP isoforms. Examples of dendritic sections from two different neurons are shown for each isoform. GFP (green) and SynGAP labelling (red) are shown above the overlaid images. Scale bar, 2 μm. Dendritic protein expression levels of various SynGAP isoforms expressed in SynGAP −/− neurons were quantified by semi-quantitative confocal microscopy ( Supplementary Fig. S2 ). Full size image Heterogenous effect of SynGAP isoforms on mEPSC amplitudes We next investigated the characteristics of functional synaptic activity in cells that exhibited detectable mEPSCs. Owing to the signal-to-noise ratio and finite duration of a recording, it is impossible to conclude that mEPSCs are completely absent from nominally 'silent' cells. In other words, the data could be censored, both by the amplitude detection threshold (5 pA) and the duration of the initial analysis period (2 min in each case, corresponding to an event frequency of 0.0083 Hz). Previous work has attempted to estimate the population amplitude and frequency by setting the values for 'silent' cells to their respective censorship bounds [19] . We have performed a similar analysis to that described by Milstein and Nicoll [19] and this is shown in Supplementary Fig. S3 . However, there are two drawbacks to this approach: first, it strongly biases the estimates of the population means; second, it will lead to an underestimate of the variance and invalidate the interpretation of statistical tests. For these reasons, and owing to the observation that our non-silent cell data are distributed well away from the censorship bounds (>2 standard deviations for mEPSC amplitude and >5 standard deviations for log frequency, Supplementary Fig. S4 ), we decided not to include threshold values for silent cells in subsequent analyses. To examine the amplitude and frequency of transfected cells in which mEPSCs were detected, we developed a statistical analysis that takes into account the potentially confounding effects of pooling data from different transfections and culture batches; specifically we used a generalized linear mixed model (GLMM) with transfection batch and culture batch as random effects ( Supplementary Information ). In addition to introducing a silencing effect, the mean mEPSC amplitude (in those cells where such events were present) also showed a dependency on the SynGAP isoform that was expressed ( Fig. 6a ). The mean mEPSC amplitude ( Fig. 6b ) of SynGAP Aα1-expressing neurons (15.6 pA) is decreased relative to control (22.3 pA). In addition, mean mEPSC amplitude was elevated in SynGAP Bα2- and Cα2-expressing neurons (26.9 and 27.8 pA, respectively, Fig. 6b ) but not in SynGAP Aα2-expressing neurons (21.8 pA). Taken together, these results suggest that SynGAP α2 is capable of positively regulating synaptic strength, but this function is dependent on its N-terminal identity (F (6, 116) =4.69, P <0.001, linear mixed model (LMM)). 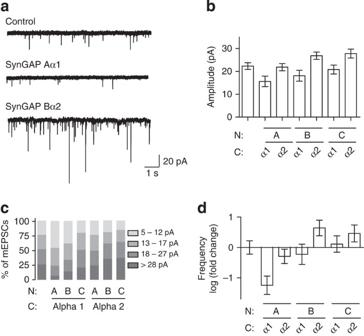Figure 6: Effects of the expression of different N- and C-termini combinations on mEPSCs. (a) Representative traces from neurons expressing SynGAP isoforms. (b) Mean mEPSC amplitudes from non-silent neurons transfected with different SynGAP isoforms. Data are displayed as a population mean of cell means (~300 mEPSC events per cell) ±s.e.m. (F(6, 116)=4.69,P<0.001, LMM). Mean mEPSC amplitudes (pA±s.e.m.) are control=22.3±1.5, Aα1=15.6±2.3, Aα2=21.8±1.6, Bα1=18.1±2.4, Bα2=26.8±1.6, Cα1=20.8±1.9 and Cα2=27.8±1.9. (c) Distribution of all mEPSCs recorded from non-silent neurons transfected with each SynGAP isoforms was classified into four amplitude categories based on the quartiles of the control population of events. (d) Frequency of mEPSCs recorded from non-silent neurons transfected with different SynGAP isoforms. Data were log transformed in order to make their distribution approximately Gaussian (Methods) and are expressed relative to control thus representing log (fold change) of mEPSC frequency (F(6, 97)=5.96,P<0.001, LMM, ±s.e.m.). Absolute mEPSC frequencies (Hz±SEM) are control=2.07±1.24, Aα1=0.6±1.35, Aα2=1.55±1.26, Bα1=1.65±1.39, Bα2=3.94±1.29, Cα1=2.32±1.3 and Cα2=3.29±1.32. Figure 6: Effects of the expression of different N- and C-termini combinations on mEPSCs. ( a ) Representative traces from neurons expressing SynGAP isoforms. ( b ) Mean mEPSC amplitudes from non-silent neurons transfected with different SynGAP isoforms. Data are displayed as a population mean of cell means (~300 mEPSC events per cell) ±s.e.m. (F (6, 116) =4.69, P <0.001, LMM). Mean mEPSC amplitudes (pA±s.e.m.) are control=22.3±1.5, Aα1=15.6±2.3, Aα2=21.8±1.6, Bα1=18.1±2.4, Bα2=26.8±1.6, Cα1=20.8±1.9 and Cα2=27.8±1.9. ( c ) Distribution of all mEPSCs recorded from non-silent neurons transfected with each SynGAP isoforms was classified into four amplitude categories based on the quartiles of the control population of events. ( d ) Frequency of mEPSCs recorded from non-silent neurons transfected with different SynGAP isoforms. Data were log transformed in order to make their distribution approximately Gaussian (Methods) and are expressed relative to control thus representing log (fold change) of mEPSC frequency (F (6, 97) =5.96, P <0.001, LMM, ±s.e.m.). Absolute mEPSC frequencies (Hz±SEM) are control=2.07±1.24, Aα1=0.6±1.35, Aα2=1.55±1.26, Bα1=1.65±1.39, Bα2=3.94±1.29, Cα1=2.32±1.3 and Cα2=3.29±1.32. Full size image The differences between the distributions of mEPSCs amplitudes are also illustrated if the quartiles of the control population (as was shown in Fig. 4d ) are plotted in the absence of silent neurons ( Fig. 6c ). The distributions of mEPSC amplitudes from SynGAP Aα1- and Bα1-expressing cells showed a larger proportion of events within the smallest amplitude range of 5–12 pA (46% and 39%, respectively). Accordingly, the largest amplitude range of >28 pA contained a smaller proportion of SynGAP Aα1 and Bα1 events (7% and 14%, respectively). The frequency distributions of mEPSC amplitudes for neurons transfected with all SynGAP isoforms, except SynGAP Aα2, were significantly different from that of eGFP-transfected control neurons ( Supplementary Fig. S5 ). Heterogenous effect of SynGAP isoforms on mEPSC frequency mEPSC frequency reflects the total number of functional synapses on a cell. We examined the mEPSC frequencies of non-silent cells by calculating the mean inter-event-interval for each cell. Consistent with their effect on silencing and event amplitude, SynGAP isoforms were also found to influence mEPSC event frequency ( Fig. 6d , F (6, 97) =5.96, P <0.001, LMM). Mean event frequencies for control cells were 2.1 Hz while SynGAP Aα1 showed a diminished event frequency of 0.6 Hz. SynGAP Bα2-expressing cells exhibited an increase in mEPSC frequency (3.9 Hz) when compared with either eGFP-only or SynGAP Aα2-expressing neurons (2.1 and 1.6 Hz, respectively). SynGAP Aα1 does not alter dendritic spine density, width or length SynGAP Aα1 showed the greatest effect on neuronal silencing with 72.5% of transfected neurons showing no detectable mEPSCs. To determine whether this silencing resulted from an inability of these neurons to form postsynaptic specializations, we examined spine density and spine morphology in SynGAP Aα1-transfected cells compared with GFP-transfected cells. We found no difference in any parameter examined ( Fig. 7 ), indicating that the silencing of hippocampal neurons by SynGAP Aα1 does not result from the loss or altered morphology of the postsynaptic apparatus despite the clear localization of this isoform to spines (see Fig. 5 ). 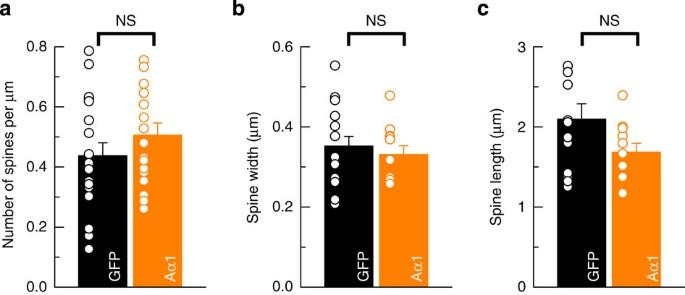Figure 7: Dendritic spine density and morphology are not altered in SynGAP Aα1 transfected neurons. No significant differences are observed between GFP- or Aα1-transfected neurons in spine density (GFP,n=20, Aα1,n=19) (a), spine width (GFP,n=16, Aα1,n=11) (b) or spine length (GFP,n=16, Aα1,n=11) (c) indicating that the silencing of hippocampal neurons by SynGAP Aα1 does not result from the loss or altered morphology of the postsynaptic apparatus. Error bars represent s.e.m. NS, nonsignificant. Figure 7: Dendritic spine density and morphology are not altered in SynGAP Aα1 transfected neurons. No significant differences are observed between GFP- or Aα1-transfected neurons in spine density (GFP, n =20, Aα1, n =19) ( a ), spine width (GFP, n =16, Aα1, n =11) ( b ) or spine length (GFP, n =16, Aα1, n =11) ( c ) indicating that the silencing of hippocampal neurons by SynGAP Aα1 does not result from the loss or altered morphology of the postsynaptic apparatus. Error bars represent s.e.m. NS, nonsignificant. Full size image Syngap is a complex gene that gives rise to numerous protein products. Little was known, however, about whether these distinct isoforms vary in expression profiles and/or function. Using 5′ RACE, we found that the variation in amino-acid sequence at the N-terminus of SynGAP (SynGAP A, B and C) arises from alternative promoter usage, with each 5′ variant showing a distinct profile of activity-dependent and developmental expressions. Furthermore, we show that SynGAP function is determined by the unique combination of N- and C-terminal domains. Previous work on SynGAP focused exclusively on the α1 C-terminus and showed that its expression led to the weakening of synaptic strength. We demonstrate that expression of a different C-terminus, α2, can lead to the opposing effect of synaptic strengthening. The magnitude of the effect in both cases was determined by the identity of the N-terminus of the protein: SynGAP Aα1 showed the largest synaptic weakening effect and SynGAPs Bα2 and Cα2 strengthened the synapse while Aα2 had no effect. These findings illustrate a novel mechanism whereby alternative promoter usage and alternative splicing combine to regulate synaptic function ( Fig. 8 ). 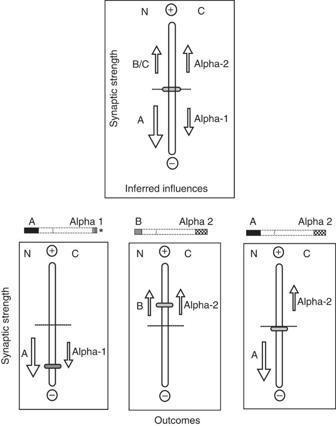Figure 8: Summary of the combinatorial effects of SynGAP N- and C-termini on synaptic strength. A slider scale is used to illustrate the effect of SynGAP isoforms on synaptic strength. The control synaptic strength is indicated with a dashed line, increased synaptic strength (+) and decreased synaptic strength (−). We can infer the influences of each individual component, or terminus, illustrated in the upper panel. The lower panels show the examples of individual isoforms as determined by the experiments in this paper. N-termini B and C are combined due to their similar, but not identical, effects. A larger arrow is used for SynGAP A to show that its influence may be stronger than that of the other regions. Figure 8: Summary of the combinatorial effects of SynGAP N- and C-termini on synaptic strength. A slider scale is used to illustrate the effect of SynGAP isoforms on synaptic strength. The control synaptic strength is indicated with a dashed line, increased synaptic strength (+) and decreased synaptic strength (−). We can infer the influences of each individual component, or terminus, illustrated in the upper panel. The lower panels show the examples of individual isoforms as determined by the experiments in this paper. N-termini B and C are combined due to their similar, but not identical, effects. A larger arrow is used for SynGAP A to show that its influence may be stronger than that of the other regions. Full size image On stimulation of synaptic activity, we found no change in total Syngap mRNA, however, the relative abundance of the various N-terminal isoforms were altered. These findings suggest that all three N-terminal isoforms are under distinct, but possibly overlapping, transcriptional control. As N-terminal isoform expression alters the synaptic function of SynGAP, synaptic activity not only controls synaptic function through transcriptional control of protein levels, but also by regulating the isoform expression through the use of alternative promoters. Activity-dependent regulation of alternative promoter usage has been reported for Bdnf , but unlike Syngap , this regulation does not alter the BDNF protein [20] . Although functional diversity of activity-regulated alternative splicing-derived isoforms is well established [3] , [21] , we know of no example where activity-regulated alternative promoter usage gives rise to protein isoforms with different, let alone opposing, effects on synaptic function. Our data indicate that the functional consequences of changes in Syngap transcription can vary depending on the promoter being used and, hence, the isoform expressed. Little is known about the transcription factors that regulate Syngap expression but examination of ENCODE data highlights two chromosomal regions that are likely to be involved. Future experiments will be necessary to determine the precise promoter elements and transcription factors that regulate the developmental and activity-dependent expression of particular SynGAP isoforms. In addition to N-terminal variation, several C-terminal isoforms of SynGAP have been described. The most studied isoforms contain the α1 C-terminus, which contains the PDZ-binding motif (QTRV) responsible for SynGAP's binding to scaffolding proteins such as PSD-95 and SAP-102. Rumbaugh et al . [6] observed a 50% decrease in mEPSC amplitude and an 85% decrease in mEPSC frequency in neurons overexpressing SynGAP Cα1; no alteration in synaptic function was seen if the last residue of the PDZ-binding domain (QTRV/E) was mutated. We also find that SynGAP α1 negatively regulates synaptic transmission, both increasing the proportion of silent cells and decreasing amplitude and frequency of remaining mEPSCs. We found that SynGAP Aα1 had the largest effects, silencing 72.5% of transfected neurons, whereas Bα1- and Cα1-containing isoforms approximately 45% of neurons. In contrast, Syngap Bα2 and Cα2 led to an increase in synaptic strength indicating that the direction of synaptic modulation exerted by SynGAP is dependent on the isoform in question ( Fig. 8 ). Our mass spectrometry analysis, locating both α1 and α2 at synapses, also supports previous findings showing that SynGAP isoforms lacking a functional PDZ-binding domain localize to synapses [6] , indicating that there are multiple microdomains with which SynGAP can associate to regulate synaptic function. The ability of SynGAP α2 to increase mEPSC amplitude and frequency is dependent on the N-terminal peptide sequence as SynGAP Bα2 increased both parameters, but SynGAP Aα2 did not alter synaptic function. Clearly, the knowledge of which isoforms, where and in what amounts is key to understanding the physiological role of SynGAP. However, similar to other extensively spliced molecules, it is likely that all combinations of all N- and C-terminal combinations exist [22] . This study illustrates that the full peptide sequence of a protein, N- terminus to C-terminus, and combinations thereof, must be considered when examining its functional properties. Our findings likely explain several discrepancies in the literature showing that SynGAP can act as both a negative and a positive regulator of synaptic strength. For example, reduction of SynGAP expression has been seen to both increase [7] and decrease [9] the synaptic expression of AMPA receptors. This apparent contradiction could be explained by findings that SynGAP can be a RasGAP and negatively regulate the ERK/MAPK pathway to reduce the synaptic delivery of AMPA receptors, but can also be a RapGAP negatively regulating the p38/MAPK pathway to prevent the removal of synaptic AMPA receptors [23] . Crucially, regions outwith the GAP domain have been shown to be essential in allowing SynGAP, and other bifunctional GAPs, to work as RapGAPs (ref. 24 and references within). Further work is required to determine whether different SynGAP isoforms differ in their Ras/Rap specificity and whether this is a mechanism by which SynGAP exerts opposing effects on synaptic strength. Alternatively, the reduction in mEPSC frequencies could result from changes in presynaptic release probability. Our low transfection efficiency means that a negligible percentage of inputs arise from other transfected neurons, making it unlikely that presynaptic expression of SynGAP causes the 'silencing'. Furthermore, the normal density and morphology of dendritic spines suggests the 'silencing' effect of SynGAP Aα1 is not the result of a large-scale loss of postsynaptic machinery. Alterations in presynaptic function could result from retrograde signalling between transfected (postsynaptic) neurons and presynaptic release sites. Alternatively, recent studies have suggested that AMPA receptor populations activated by spontaneous (TTX-insensitive) and evoked (action potential dependent) release of glutamate may be distinct [25] . Therefore, isoforms of SynGAP may differentially regulate the distribution of glutamate receptors within the postsynaptic membrane. Irrespective of how SynGAP alters synaptic function, our findings indicate that the regulation of expression of a single gene, Syngap , through the combination of alternative promoter usage and splicing can markedly alter the function of the resulting protein. Understanding the mechanisms by which synaptic plasticity is induced and expressed is key to our understanding of brain development as well as adult learning and memory. We demonstrate that the expression of multiple protein isoforms from a single gene can have opposing effects on synaptic function. Although functional diversity among activity-dependent alternatively spliced isoforms is well established [3] , each SynGAP isoform has a unique effect on synaptic function that is determined by the combination of the N- and C-termini that results from the use of multiple alternative promoters and alternative splicing, respectively. This creates an exquisitely fine-tuned system that allows synaptic activity and developmental stage to alter protein isoform expression to control not only the magnitude, but also crucially the direction, of synaptic plasticity. Molecular biology 5′ RACE was performed on RNA isolated from p14 forebrain of C57Bl6 mice (FirstChoice RLM-RACE kit). Quantitative RT–PCR was performed using RNA isolated from forebrain and stimulated neuronal culture lysates using primers complementary to Syngap variant-specific sequences and normalized to 18S rRNA or glyceraldehyde 3-phosphate dehydrogenase mRNA expression. Full-length SynGAP Aα2 was isolated from Superscript Mouse Brain plasmid cDNA library (10655025 in pCMV-sport6, Invitrogen) by colony hybridization using a 32 P-dCTP-labelled DNA probe specific to a central region of SynGAP. The range of SynGAP clones used were then constructed from this clone, a separately isolated SynGAP α1 clone and 5′ regions of B and C, which were cloned by PCR amplification from forebrain cDNA, and subcloned without 3′ UTR into a cytomegalovirus expression vector. Additional details, including construction specifics and primer sequences, are given in the Supplementary Information . Identification of SynGAP isoforms by mass spectrometry In order to validate the presence of SynGAP isoforms in the PSD, tandem mass spectrometry data obtained from analysis of purified mouse PSD and PSD-95-associated complexes [26] , [27] were analysed for the presence of isoform-specific sequences. Briefly, tandem mass spectrometry data were processed using Proteome Discoverer version 1.1 (Thermo Fisher Scientific) and the resultant peak lists were searched against a mouse IPI database (downloaded June 2007) supplemented with SynGAP isoform sequences using MASCOT v2.2 (Matrix science). Precursor ion tolerance was set to 10 p.p.m. and fragment ion tolerance was set to 0.5 Da. Enzyme specificity was set to Trypsin with two missed cleavages. Carbamidomethyl modification of cysteine residues, oxidation of methionine, deamidation of asparagine and glutamine residues and acetyl (protein N-term) were set as variable modifications. The Mascot search results were then submitted to our in-house version of Mascot Percolator v1.1 to re-score peptide spectrum matches and to produce a final set of peptide identifications with a 1% (peptide level) false discovery rate. Tandem mass spectra that identified SynGAP isoform-specific sequences ( Supplementary Data 1 ) were manually inspected. See Supplementary Table S2 for representative spectra and Supplementary Methods for a link to the appropriate database. Neuronal cultures Mouse forebrain cultures were derived from E17.5 embryos and maintained in Neurobasal, B-27, Glutamax, Pen/Strep (Invitrogen). Cultured neurons (days in vitro (DIV) 10–12) were stimulated with Bic (50 μM) and 4-AP (250 μM) to induce an increase in the frequency of action potential-evoked synaptic currents [28] . Biochemistry For comparison of SynGAP isoform molecular weights, mouse P14 brain lysates were electrophoresed in a single large well, transferred to nitrocellulose, cut into strips and probed with isoform-specific SynGAP antibodies; pan (Cambridge Biosciences, PA-046, 1:4,000), α1 (Millipore, 06-900, 1:4,000), α2 (Abcam, EPR2883Y, 1:4,000). Quantification was performed by densitometry (ImageJ) and normalized against Neurofilament M (Abcam, Cambridge, MA, USA, 1:6,000), similar results we obtained by normalization against β-actin (Abcam, 1:10,000). Standard western blotting was completed as previously described [17] . Electrophysiology Whole-cell patch-clamp recordings were performed on DIV 9–11 fluorescent neurons between 16 and 36 h after liposome-mediated co-transfection with eGFP and SynGAP. External recording solution contained (in mM) NaCl (150), KCl (3), HEPES (10), Glucose (10), CaCl 2 (2.5), MgCl 2 (1.3), pH 7.3. Internal solution contained (in mM) K-gluconate (130), KCl (10), HEPES (10), EGTA (0.1), glucose (10), Na-phosphocreatine (10), Mg-ATP (4), Mg-GTP (0.5), pH 7.3. mEPSCs were recorded at a holding potential of −70 mV in the presence of TTX (500 nM) and picrotoxin (50 μM). Access resistance (Ra) was monitored following membrane rupture and dialysis, and recordings were abandoned if Ra >28 MΩ. Recordings with an unstable or >−150 pA holding current or high noise (greater than 4 pA root mean square (RMS)) were excluded. For mEPSC analysis, at least 6 min of spontaneous activity was recorded from each cell, with access resistance measured every 2 min. An event amplitude threshold was set at 5 pA above the baseline, at least 300 events were analysed per cell. A minimum recording length of 2 min, where no mEPSCs were apparent, was required for a cell to be classified as silent. No minimum recording length was necessary to designate a cell as non-silent, the appearance of obvious mEPSCs was sufficient. Cells with high RMS noise but with mEPSCs obvious above the noise were not included in this analysis. Statistical analysis mEPSC amplitude and frequency data from the SynGAP overexpression experiments ( Fig. 4 ) were analysed by fitting a LMM using residual maximum likelihood in GenStat v13 (VSN International). Data fitted in the model represented mean event amplitudes and (log) event frequencies for individual cells (123 'non-silent' cells, 15 culture batches and 18 transfections). Culture batch (representing cells from the same tissue) and Transfection (representing repeat transfections) were included in the model as random effects, with no interaction term; the fixed effect was the Expression Construct (levels=GFP, SynGAP Aα1 and so on). Residuals were examined to check for the appropriateness of the normality assumption and revealed a satisfactory fit ( Supplementary Fig. S6 ). The proportions of silent cells observed were analysed similarly ( Fig. 4 ), using a GLMM with a binomial data model (allowing for under/overdispersion) and a logit link function (218 cells, 15 culture batches and 18 transfections). Again, Expression Construct was included as a fixed effect, whereas Culture batch and Transfection were included as random effects, with no interaction term. F-statistics represent Wald tests between the full model and a model in which the fixed effect is dropped. Model output is included for both LMMs and the GLMM in the Supplementary Information . Informations on other statistical tests used are found within the relevant figure legends. How to cite this article: McMahon, A. C. et al . SynGAP isoforms exert opposing effects on synaptic strength. Nat. Commun. 3:900 doi: 10.1038/ncomms1900 (2012).